Loss of PIKfyve in platelets causes a lysosomal disease leading to inflammation and thrombosis in mice PIKfyve is essential for the synthesis of phosphatidylinositol-3,5-bisphosphate [PtdIns(3,5)P 2 ] and for the regulation of endolysosomal membrane dynamics in mammals. PtdIns(3,5)P 2 deficiency causes neurodegeneration in mice and humans, but the role of PtdIns(3,5)P 2 in non-neural tissues is poorly understood. Here we show that platelet-specific ablation of PIKfyve in mice leads to accelerated arterial thrombosis, and, unexpectedly, also to inappropriate inflammatory responses characterized by macrophage accumulation in multiple tissues. These multiorgan defects are attenuated by platelet depletion in vivo , confirming that they reflect a platelet-specific process. PIKfyve ablation in platelets induces defective maturation and excessive storage of lysosomal enzymes that are released upon platelet activation. Impairing lysosome secretion from PIKfyve-null platelets in vivo markedly attenuates the multiorgan defects, suggesting that platelet lysosome secretion contributes to pathogenesis. Our findings identify PIKfyve as an essential regulator for platelet lysosome homeostasis, and demonstrate the contributions of platelet lysosomes to inflammation, arterial thrombosis and macrophage biology. Phosphoinositides are minor components of membrane phospholipids, yet they are essential for the regulation of diverse cellular processes, including signal transduction, cytoskeletal control and membrane trafficking [1] . Phosphoinositide metabolism is tightly modulated by specific lipid kinases and phosphatases. Altering phosphoinositide turnover by dysregulating these enzymes can lead to a variety of human diseases [2] . PtdIns(3,5)P 2 is a phosphoinositide of low abundance that is synthesized from PtdIns(3)P on the endosomal compartments in mammalian cells by the lipid kinase PIKfyve (also known as FAB1) [3] . PIKfyve forms a protein complex with other regulatory proteins, such as the PtdIns(3,5)P 2 5-phosphatase Fig4 (also known as SAC3) [4] , [5] and the docking protein Vac14 (also known as ArPIKfyve) [6] , [7] . The PIKfyve complex and its product PtdIns(3,5)P 2 are essential regulators of membrane homeostasis, and of vesicle trafficking and cargo transport along the endosomal–lysosomal pathway [8] , [9] . Recently, physiological functions of PtdIns(3,5)P 2 have been elucidated using genetically engineered mice that lack different components of the PIKfyve complex [10] . PIKfyve-null mice are embryonically lethal [11] , but mice expressing residual PIKfyve activity are viable and develop defects within multiple organs, such as in the nervous, cardiopulmonary and hematopoietic systems [12] . Similarly, Fig4-null mice or Vac14-null mice develop several defects, including neurodegeneration, hypopigmentation and early lethality [13] , [14] . Notably, homozygous Fig4 mutations were also identified in patients who have the neurodegenerative diseases Charcot–Marie–Tooth syndrome 4J and amyotrophic lateral sclerosis [14] , [15] , demonstrating a role for PtdIns(3,5)P 2 in neural development. Although studies showed that PtdIns(3,5)P 2 deficiency causes defects in multiple cellular pathways including those required for endolysosomal trafficking in yeast and mammalian cell cultures, the physiological consequences of PtdIns(3,5)P 2 in non-neural cells, such as those of the hematopoietic system, are not well understood. Platelets are hematopoietic cells that are crucial for haemostatic plug formation in response to vascular injury. This process has been shown to require a series of key platelet activation events that are tightly regulated by several phosphoinositides [16] . However, the regulatory role of PtdIns(3,5)P 2 in platelets remains unknown. Platelets are anucleated, but they store numerous biologically active substances in their secretory organelles, which include alpha granules, dense granules and lysosomes [17] , [18] . Platelet granules are generated in megakaryocytes from the endosomal–lysosomal system [19] , [20] , [21] , [22] by, as yet, poorly understood mechanisms. In this study, we investigated whether PIKfyve has an essential role in platelets and in megakaryocytes using mice lacking PIKfyve specifically in these cell types. Given the role of PIKfyve-mediated PtdIns(3,5)P 2 production in the regulation of the endosomal–lysosomal pathway, we hypothesized that PIKfyve was essential for the biogenesis and function of platelet granules. We show that PIKfyve is critical for proper lysosomal homeostasis in platelets, but it is not necessary for the biogenesis of alpha granules or dense granules. Remarkably, PIKfyve-null platelets are defective in the maturation, storage and release of lysosomal enzymes. Unexpectedly, these platelet lysosomal defects induce aberrant inflammatory responses in macrophages that impair the development, body mass, fertility and survival of mice. Loss of PIKfyve in platelets causes multiorgan defects To investigate the role of PIKfyve in platelets and in megakaryocytes, we generated mice lacking PIKfyve kinase activity specifically in these cell types. The PIKfyve gene was conditionally targeted with loxP sites flanking the exons corresponding to the kinase activation loop to generate floxed alleles of PIKfyve ( PIKfyve fl , Fig. 1a ). Mice expressing PIKfyve fl were crossed with transgenic mice expressing the Cre recombinase that is controlled by the platelet-factor-4 promoter ( Pf4-Cre ), which restricts the expression of Cre recombinase exclusively within megakaryocytes and their derived platelets [23] . 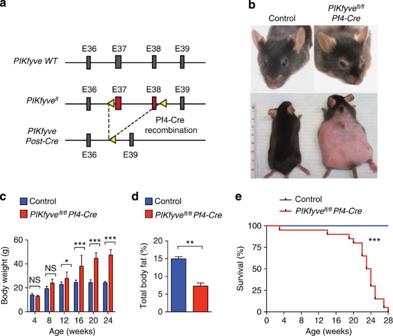Figure 1: Platelet-specific ablation of PIKfyve causes multiorgan abnormalities in mice. (a) Schematic representation of genetic targeting ofPIKfyve. The target exons 37 and 38 (red bars) were targeted with lox P recombination sites (yellow arrows) to generatePIKfyve-floxed alleles (PIKfyvefl). Mice expressingPIKfyveflwere then crossed withPf4-Cremice to induce homologous recombination of thePIKfyvefl(PIKfyve Post-Cre). (b) General appearance of control andPIKfyvefl/flPf4-Crelittermates at 24 weeks of age. Note the characteristic coarse facial features, body hair loss and severely distended body morphology. (c) Body weight of control mice andPIKfyvefl/flPf4-Cremice. The average numbers of mice were eight per time point and per group. (d) Percent of total body fat in the control (n=3) andPIKfyvefl/flPf4-Cre(n=3) mice at 12–24 weeks of age. (e) Survival curves of female and male control (n=40) andPIKfyvefl/flPf4-Cre(n=40) mice. *P<0.05, **P<0.01, ***P<0.001. All error bars indicate mean±s.d. Student’st-test. Figure 1: Platelet-specific ablation of PIKfyve causes multiorgan abnormalities in mice. ( a ) Schematic representation of genetic targeting of PIKfyve . The target exons 37 and 38 (red bars) were targeted with lox P recombination sites (yellow arrows) to generate PIKfyve -floxed alleles ( PIKfyve fl ). Mice expressing PIKfyve fl were then crossed with Pf4-Cre mice to induce homologous recombination of the PIKfyve fl ( PIKfyve Post-Cre ). ( b ) General appearance of control and PIKfyve fl/fl Pf4-Cre littermates at 24 weeks of age. Note the characteristic coarse facial features, body hair loss and severely distended body morphology. ( c ) Body weight of control mice and PIKfyve fl/fl Pf4-Cre mice. The average numbers of mice were eight per time point and per group. ( d ) Percent of total body fat in the control ( n =3) and PIKfyve fl/fl Pf4-Cre ( n =3) mice at 12–24 weeks of age. ( e ) Survival curves of female and male control ( n =40) and PIKfyve fl/fl Pf4-Cre ( n =40) mice. * P <0.05, ** P <0.01, *** P <0.001. All error bars indicate mean±s.d. Student’s t -test. Full size image PIKfyve fl/fl Pf4-Cre mice developed several morphological abnormalities relative to their littermate PIKfyve fl/+ mice, PIKfyve fl/fl mice and PIKfyve fl/+ Pf4-Cre mice. At about 3 weeks of age, PIKfyve fl/fl Pf4-Cre mice exhibited mild growth delay and body hair loss ( Supplementary Fig. 1a ). Over time, they gradually developed coarse facial features, abdominal distention, a generalized increase in the bulk of their soft tissues and body weight gain ( Fig. 1b,c ). Despite this weight gain, body composition analysis by dual-energy X-ray absorptiometry showed that PIKfyve fl/fl Pf4-Cre mice had reduced body fat, but increased lean body mass, as compared with their littermate controls ( Fig. 1d ). In addition, they also had decreased bone mineral density ( Supplementary Fig. 1b ). As PIKfyve fl/fl Pf4-Cre mice aged, they remained infertile ( Supplementary Fig. 1c ) and their general body functions deteriorated. The vast majority died before 28 weeks of age ( Fig. 1e ). PIKfyve fl/fl Pf4 - Cre mice accumulate vacuolated macrophages To elucidate the cause of multiorgan defects in PIKfyve fl/fl Pf4-Cre mice, histological and immunohistochemical analyses were performed in mice of 3–28 weeks of age. Unlike their control littermates, PIKfyve fl/fl Pf4-Cre mice exhibited massive organomegaly ( Supplementary Fig. 2a ). This phenotype reflected progressive tissue infiltration by engorged cells with multiple cytoplasmic vacuoles that had a ‘foamy’ appearance ( Fig. 2a and Supplementary Fig. 2b , arrowheads). Although the vacuoles of these cells did not stain with classical dyes for proteins or lipids, their cytoplasm strongly stained with Alcian blue and periodic acid Schiff, suggesting an excessive storage of acidic polysaccharides in the vacuolated cells ( Fig. 2b and Supplementary Fig. 3a ). In their livers and lungs, the vacuolated cells accumulated in a perivascular distribution and displaced the normal tissue ( Fig. 2a ), suggesting that the vacuolated cells originated from the blood or vasculature. By immunohistochemical analysis, the vacuolated cells stained with the macrophage-specific marker F4/80 ( Fig. 2c ), but not with the markers of other cell lineages, including GPIb (a megakaryocyte-specific marker). The F4/80-positive vacuolated macrophages in the livers of PIKfyve fl/fl Pf4-Cre mice were approximately three- to fourfold larger than the F4/80-positive macrophages in the livers of the control mice ( Fig. 2d ). In addition, tissues infiltrated with the vacuolated macrophages were often associated with mononuclear cell infiltrates that stained with the lymphocyte marker CD45R ( Supplementary Fig. 3b ), suggesting a local inflammatory response. These results demonstrate that the loss of PIKfyve in platelets causes the invasion of normal tissues with inflammatory vacuolated macrophages. 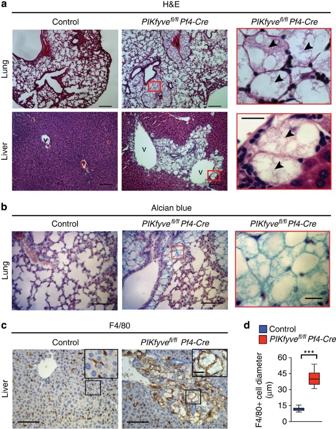Figure 2: Inflammatory vacuolated macrophages infiltrate multiple tissues in thePIKfyvefl/flPf4-Cremice. (a) Representative histological sections of the lungs and livers stained with haematoxylin and eosin (H&E) from control mice andPIKfyvefl/flPf4-Cremice. Scale bar, 100 μm. Insets show increased magnification of boxed areas ina. Scale bar, 20 μm. Arrowheads indicate the vacuolated cells. (b) Lung sections stained with Alcian blue. Scale bar, 100 μm. Inset shows high magnification of the boxed area. (c) Liver structures of control mice andPIKfyvefl/flPf4-Cremice were stained for macrophages with anti-F4/80 by immunohistochemistry. Scale bar, 100 μm. Insets in the upper right corner of each image show higher magnification images of boxed areas. Scale bar, 20 μm. (d) Cell diameters of F4/80+ cells in the livers of control mice (n=5) andPIKfyvefl/flPf4-Cremice (n=5). ***P<0.001. All error bars indicate mean±s.d. Student’st-test. Figure 2: Inflammatory vacuolated macrophages infiltrate multiple tissues in the PIKfyve fl/fl Pf4-Cre mice. ( a ) Representative histological sections of the lungs and livers stained with haematoxylin and eosin (H&E) from control mice and PIKfyve fl/fl Pf4-Cre mice. Scale bar, 100 μm. Insets show increased magnification of boxed areas in a . Scale bar, 20 μm. Arrowheads indicate the vacuolated cells. ( b ) Lung sections stained with Alcian blue. Scale bar, 100 μm. Inset shows high magnification of the boxed area. ( c ) Liver structures of control mice and PIKfyve fl/fl Pf4-Cre mice were stained for macrophages with anti-F4/80 by immunohistochemistry. Scale bar, 100 μm. Insets in the upper right corner of each image show higher magnification images of boxed areas. Scale bar, 20 μm. ( d ) Cell diameters of F4/80+ cells in the livers of control mice ( n =5) and PIKfyve fl/fl Pf4-Cre mice ( n =5). *** P <0.001. All error bars indicate mean±s.d. Student’s t -test. Full size image PIKfyve-null platelets induce macrophage pathology Cells from PtdIns(3,5)P 2 -deficient organisms have been shown to form large cytoplasmic vacuoles [9] , [10] . However, because our genetic approach was designed to only ablate PtdIns(3,5)P 2 synthesis in platelets and in megakaryocytes, we did not expect to see the robust cytoplasmic vacuolation in the macrophages of PIKfyve fl/fl Pf4-Cre mice. Therefore, we further addressed whether these unexpected macrophage abnormalities resulted from aberrant PIKfyve disruption in macrophages, or by nonautonomous effects of PIKfyve disruption in platelets. Immunoblotting analysis showed that PIKfyve protein was absent in platelets, but present in the liver, spleen and lungs of PIKfyve fl/fl Pf4-Cre mice. PIKfyve protein was also present in all tissues of the control mice ( Fig. 3a and Supplementary Fig. 4a ). These results strongly suggest that the PIKfyve protein was ablated only in the megakaryocyte lineage of PIKfyve fl/fl Pf4-Cre mice. 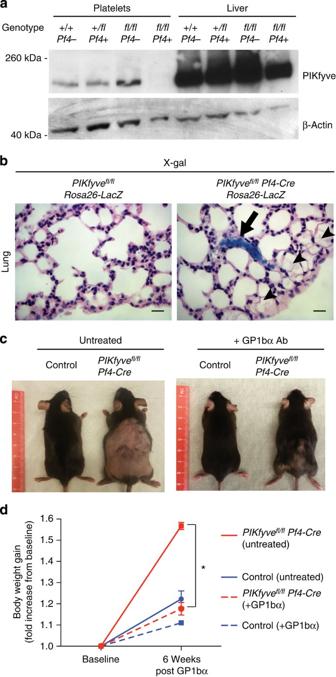Figure 3: Platelets drive the multiorgan defects in thePIKfyvefl/flPf4-Cremice. (a) The levels of PIKfyve protein were determined in the platelets and liver of the indicated mice by immunoblotting. Note the absence of the PIKfyve protein in the platelets, but its presence in the liver ofPIKfyvefl/flPf4-Cremice (n=3). Tissues from the wild-type mice, thePIKfyvefl/+Pf4-Cremice and thePIKfyvefl/flmice were used as positive controls. β-Actin was used as a loading control. (b) X-gal staining of the lung tissues fromPIKfyvefl/flRosa26-LacZmice andPIKfyvefl/flPf4-Cre Rosa26-LacZmice. Scale bar, 20 μm. The arrow indicates the platelet clumps in the lung vessels expressing LacZ (blue stain). Arrowheads indicate the vacuolated macrophages that did not stain blue. (c) Representative general morphology of 15-week-old control mice andPIKfyvefl/flPf4-Cremice after 6 weeks of either no intervention (untreated) or biweekly injections of anti-GP1bα antibodies (+GP1bα Ab). (d) Body weight change of the control mice andPIKfyvefl/flPf4-Cremice after 6 weeks of no intervention or treatment with anti-GP1bα antibodies (n=3 for each group). *P<0.05. All error bars indicate mean±s.d. Student’st-test. Figure 3: Platelets drive the multiorgan defects in the PIKfyve fl/fl Pf4-Cre mice. ( a ) The levels of PIKfyve protein were determined in the platelets and liver of the indicated mice by immunoblotting. Note the absence of the PIKfyve protein in the platelets, but its presence in the liver of PIKfyve fl/fl Pf4-Cre mice ( n =3). Tissues from the wild-type mice, the PIKfyve fl/+ Pf4-Cre mice and the PIKfyve fl/fl mice were used as positive controls. β-Actin was used as a loading control. ( b ) X-gal staining of the lung tissues from PIKfyve fl/fl Rosa26-LacZ mice and PIKfyve fl/fl Pf4-Cre Rosa26-LacZ mice. Scale bar, 20 μm. The arrow indicates the platelet clumps in the lung vessels expressing LacZ (blue stain). Arrowheads indicate the vacuolated macrophages that did not stain blue. ( c ) Representative general morphology of 15-week-old control mice and PIKfyve fl/fl Pf4-Cre mice after 6 weeks of either no intervention (untreated) or biweekly injections of anti-GP1bα antibodies (+GP1bα Ab). ( d ) Body weight change of the control mice and PIKfyve fl/fl Pf4-Cre mice after 6 weeks of no intervention or treatment with anti-GP1bα antibodies ( n =3 for each group). * P <0.05. All error bars indicate mean±s.d. Student’s t -test. Full size image Although Pf4-Cre expression has been shown to be restricted to megakaryocytes and platelets [23] , [24] , [25] , [26] , we next re-evaluated Pf4-Cre expression in PIKfyve fl/fl Pf4-Cre mice by crossing them to mice expressing a Cre-dependent LacZ reporter ( Rosa26-LacZ ) [27] . Tissue staining of PIKfyve fl/fl Pf4-Cre/Rosa26-Lacz mice with X-gal showed β-galactosidase expression only in megakaryocytes and in platelets ( Fig. 3b and Supplementary Fig. 4b , arrows), but not in the vacuolated macrophages or in the other cells ( Fig. 3b , arrowheads). This genetic evidence excludes the possibility that Pf4-Cre induced PIKfyve ablation in the macrophages of PIKfyve fl/fl Pf4-Cre mice. Together, these results demonstrate that the macrophage infiltration and enlargement observed in PIKfyve fl/fl Pf4-Cre mice are indirectly induced by PIKfyve ablation in megakaryocytes and/or in platelets. To further address whether PIKfyve-null platelets contribute to the robust macrophage response leading to the multiorgan failure in PIKfyve fl/fl Pf4-Cre mice, we studied the effects of platelet depletion using monoclonal GP1bα antibodies [28] , [29] . Platelet depletion was initiated at 8–10 weeks of age. At that point, the PIKfyve fl/fl Pf4-Cre mice had already developed body hair loss, some weight gain and tissue infiltration of their vacuolated macrophages. Control mice and PIKfyve fl/fl Pf4-Cre mice were either untreated or administered GP1bα antibodies twice weekly via intraperitoneal injections for 6 weeks. As reported previously, the injection of GP1bα antibodies efficiently induced acute thrombocytopenia in both sets of mice [28] , [29] . However, repetitive injections of GP1bα antibodies were less effective at inducing stable thrombocytopenia over time likely because of the reactive thrombocytopoiesis associated with complete platelet depletion with antiplatelet antibodies [30] . Nevertheless, the PIKfyve fl/fl Pf4-Cre mice that were treated with GP1bα antibodies showed a significant delay in weight gain and attenuated hair loss as compared with the untreated PIKfyve fl/fl Pf4-Cre mice ( Fig. 3c,d ). Together, our findings demonstrate that platelets are the primary contributors in the development of the inflammatory macrophage response and multiorgan defects in PIKfyve fl/fl Pf4-Cre mice. We also investigated whether the macrophage response in PIKfyve fl/fl Pf4-Cre mice could be rescued or transferred by hematopoietic stem cell (HSC) transplantation. Lethally irradiated wild-type mice of 8–12 weeks of age were reconstituted with a mixture of donor cells that were half derived from PIKfyve fl/fl Pf4-Cre HSCs and half derived from wild-type HSCs. Thirty-five weeks later, a necropsy showed that infiltration of vacuolated macrophages was readily apparent in the liver, lung, colon and bone marrow of the irradiated wild-type recipient mice ( Supplementary Fig. 5b,e , arrowheads). Conversely, lethally irradiated PIKfyve fl/fl Pf4-Cre mice of 8–12 weeks of age were reconstituted exclusively with wild-type donor HSCs. At about 8 weeks after transplantation, the characteristic hair loss and weight gain were significantly attenuated. A necropsy at 35 weeks after transplantation confirmed that the infiltration of the vacuolated macrophages in multiple tissues was completely reversed ( Supplementary Fig. 5c,f ). Together, these results further demonstrate that the phenotype of PIKfyve fl/fl Pf4-Cre mice can be either rescued or transferred by hematopoietic progenitor cells. Megakaryopoiesis and thrombopoiesis do not require PIKfyve We next studied the effects of PIKfyv e ablation in megakaryocytes of PIKfyve fl/fl Pf4-Cre mice. Fibroblasts and neurons of PtdIns(3,5)P 2 -deficient organisms typically develop large vacuoles [9] , [10] . Histological analysis by light microscopy of bone marrow sections showed that PIKfyve-null megakaryocytes were morphologically indistinguishable from control megakaryocytes ( Supplementary Fig. 6a ). However, analysis by transmission electron microscopy of cultured megakaryocytes derived from PIKfyve fl/fl Pf4-Cre bone marrow revealed multiple enlarged cytoplasmic vacuoles ( Fig. 4a ). Despite this abnormality, flow cytometric analysis showed no significant differences in the number of megakaryocytes in the bone marrow of control or PIKfyve fl/fl Pf4-Cre mice ( Fig. 4b ). Moreover , PIKfyve-null megakaryocytes had normal ploidy, implying that the loss of PIKfyve did not affect megakaryocyte maturation ( Fig. 4c ). Finally, counts of platelets and leukocytes as well as haemoglobin level were similar between control and PIKfyve fl/fl Pf4-Cre mice ( Fig. 4d–f ). Thus, PIKfyve fl/fl Pf4-Cre mice normally develop megakaryocytes in vivo and produce normal numbers of platelets, and they also normally develop other blood cells. 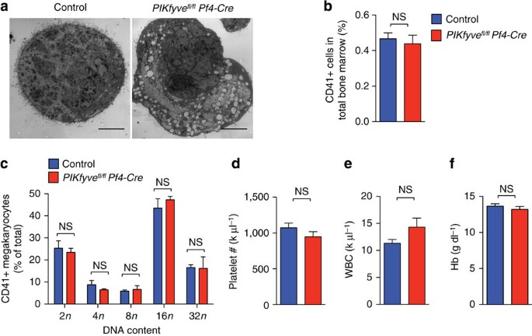Figure 4: PIKfyve is not necessary for the development of megakaryocytes nor for platelet production. (a) Electron micrographs of megakaryocytes grown in culture in the presence of thrombopoietin for 7 days. Note multiple enlarged vacuoles in the cytoplasm ofPIKfyvefl/flPf4-Cremice as compared with the control mice. Scale bar, 10 μm. (b) CD41+ megakaryocyte counts of controlPIKfyvefl/flPf4-Cremice (n=3 for each group). (c) Megakaryocyte ploidy (n=3 for each group). (d–f) Counts of platelets (d), WBC (e) and Hb (f) of control mice andPIKfyvefl/flPf4-Cremice (n=3 for each group). All error bars indicate mean±s.d. Student’st-test. Figure 4: PIKfyve is not necessary for the development of megakaryocytes nor for platelet production. ( a ) Electron micrographs of megakaryocytes grown in culture in the presence of thrombopoietin for 7 days. Note multiple enlarged vacuoles in the cytoplasm of PIKfyve fl/fl Pf4-Cre mice as compared with the control mice. Scale bar, 10 μm. ( b ) CD41+ megakaryocyte counts of control PIKfyve fl/fl Pf4-Cre mice ( n =3 for each group). ( c ) Megakaryocyte ploidy ( n =3 for each group). ( d – f ) Counts of platelets ( d ), WBC ( e ) and Hb ( f ) of control mice and PIKfyve fl/fl Pf4-Cre mice ( n =3 for each group). All error bars indicate mean±s.d. Student’s t -test. Full size image PIKfyve regulates trafficking of platelet lysosomal cargoes We next investigated the effects of PIKfyve ablation in the morphology and functions of platelets in PIKfyve fl/fl Pf4-Cre mice. Transmission electron microscopy demonstrated that in contrast to the PIKfyve-null megakaryocytes derived from the bone marrow, the ultrastructure of PIKfyve-null platelets was indistinguishable from that of control platelets ( Supplementary Fig. 6b ). To test whether the loss of PIKfyve impacted granule content, we assessed the abundance of representative components by immunoblotting. PIKfyve-null platelets expressed normal levels of the alpha granule components von Willebrand factor and platelet factor 4 ( Supplementary Fig. 6c,d ). In contrast, PIKfyve-null platelets exhibited increased levels of the lysosomal protein LAMP-1 (lysosomal-associated membrane protein 1; Fig. 5a ) and increased activity of the lysosomal enzyme β-hexosaminidase ( Fig. 5b ). These results suggest that PIKfyve-null platelets store normal levels of alpha granule components, but store excessive levels of lysosomal components. 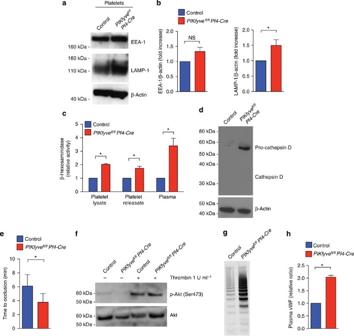Figure 5:PIKfyveis critical for the maturation, storage and release of lysosomal enzymes in platelets. (a) Immunoblot of platelet lysates from the control mice andPIKfyvefl/flPf4-Cremice showing the expression of EEA-1 and LAMP-1. β-Actin was used as the loading control. (b) Quantification of protein bands shown ina(n=3 for each group). (c) β-hexosaminidase activity in the platelet lysates, platelet relesates, and plasma of control mice (n=3) andPIKfyvefl/flPf4-Cre mice (n=3). (d) Immunoblot of platelet lysates from control mice andPIKfyvefl/flPf4-Cremice showing the expression of Procathepsin D. β-actin was used as the loading control. (e) Time to occlusion of carotid arteries upon vascular injury with 7.5% of FeCl3in the control mice (n=9) and thePIKfyvefl/flPf4-Cremice (n=8). (f) Immunoblot of platelet lysates from control platelets andPIKfyvefl/flPf4-Creplatelets showing the Akt phosphorylation in resting condition or stimulated with 1 U ml−1of thrombin for 10 min. (g) SDS agarose electrophoresis showing the multimer pattern of plasma vWF from the control mice (n=3) and thePIKfyvefl/flPf4-Cre(n=3) mice. (h) Plasma levels of vWF from the control mice (n=3) and thePIKfyvefl/flPf4-Cre(n=3) mice were quantified by ELISA. *P<0.05. All error bars indicate mean±s.d. Student’st-test. Figure 5: PIKfyve is critical for the maturation, storage and release of lysosomal enzymes in platelets. ( a ) Immunoblot of platelet lysates from the control mice and PIKfyve fl/fl Pf4-Cre mice showing the expression of EEA-1 and LAMP-1. β-Actin was used as the loading control. ( b ) Quantification of protein bands shown in a ( n =3 for each group). ( c ) β-hexosaminidase activity in the platelet lysates, platelet relesates, and plasma of control mice ( n =3) and PIKfyve fl/fl Pf4-Cre mice ( n =3). ( d ) Immunoblot of platelet lysates from control mice and PIKfyve fl/fl Pf4-Cre mice showing the expression of Procathepsin D. β-actin was used as the loading control. ( e ) Time to occlusion of carotid arteries upon vascular injury with 7.5% of FeCl 3 in the control mice ( n =9) and the PIKfyve fl/fl Pf4-Cre mice ( n =8). ( f ) Immunoblot of platelet lysates from control platelets and PIKfyve fl/fl Pf4-Cre platelets showing the Akt phosphorylation in resting condition or stimulated with 1 U ml −1 of thrombin for 10 min. ( g ) SDS agarose electrophoresis showing the multimer pattern of plasma vWF from the control mice ( n =3) and the PIKfyve fl/fl Pf4-Cre ( n =3) mice. ( h ) Plasma levels of vWF from the control mice ( n =3) and the PIKfyve fl/fl Pf4-Cre ( n =3) mice were quantified by ELISA. * P <0.05. All error bars indicate mean±s.d. Student’s t -test. Full size image To test whether PIKfyve regulates granule secretion, we stimulated platelets ex vivo and monitored granule release by surface expression of granule markers or release of mediators into the medium. Following thrombin stimulation, PIKfyve-null platelets translocated the α-granule protein P-selectin to their cell surface as efficiently as control platelets ( Supplementary Fig. 7a ). Likewise, ATP secretion from dense granules was similar in control and PIKfyve-null platelets ( Supplementary Fig. 7b ). However, the releasates from PIKfyve-null platelets showed increased activity of the lysosomal enzyme, β-hexosaminidase ( Fig. 5c ). Further analysis showed that the PIKfyve-null platelets released a normal percentage of their total cellular β-hexosaminidase following agonist stimulation ( Supplementary Fig. 7c ). These data indicate that PIKfyve-null platelets release higher levels of β-hexosaminidase than the control platelets because they contain excessive amounts of this lysosomal enzyme, and not because they secrete it more efficiently. Consistent with this finding, β-hexosaminidase activity was found to also be elevated in the plasma of PIKfyve fl/fl Pf4-Cre mice ( Fig. 5c ). Together, these findings demonstrate that PIKfyve-null platelets store and release excessive levels of lysosomal cargo proteins. To more comprehensively analyse how the loss of PIKfyve affects the contents secreted upon platelet activation, a quantitative proteomics analysis was performed. By tandem liquid chromatography-mass spectrometry (LC-MS/MS), we identified the proteins released from the control platelets and the PIKfyve-null platelets following thrombin stimulation. We then used the spectral counting of the identified peptides to quantitatively compare the proteins released from the control platelets and the PIKfyve-null platelets. Using a cutoff of 2.0-fold as a significant difference between them, we identified 17 proteins that were increased and 38 proteins that were decreased in the releasates of PIKfyve-null platelets relative to wild-type platelets ( Supplementary Tables 1 and 2 ). Among those proteins that were more abundant in the PIKfyve-null platelet releasates, several lysosomal enzymes stood out including cathepsin D, cathepsin B and maltase ( Supplementary Table 1 ). Remarkably, levels of the cathepsin D were 20-fold higher in PIKfyve-null platelet releasates than in control releasates ( Supplementary Table 1 ). Further analysis of the sequence coverage and MS spectra of the tryptic peptides for cathepsin D demonstrated that the releasates of PIKfyve-null platelets contained predominantly the procathepsin D—the immature and inactive proenzyme form of cathepsin D—but undetectable levels of mature cathepsin D ( Supplementary Fig. 8a–c ). To further validate these findings, we analysed the expression of cathepsin D in platelet lysates by immunoblotting. Consistent with the proteomics data, both cathepsin D and procathepsin D were undedetectable in the lysates of wild-type platelets, and procathepsin D was highly elevated in PIKfyve-null platelets ( Fig. 5d ). These results suggest that cathepsin D expression is upregulated in PIKfyve-null platelets, but that the intracellular maturation of procathepsin D is defective in PIKfyve-null platelets. Consequently, cathepsin D activity was negligible in both the lysates and releasates of both wild-type and the PIKfyve-null platelets ( Supplementary Fig. 7d ). Together, these data demonstrate that PIKfyve ablation in platelets results in a defective lysosomal pathway reflected by abnormal storage, maturation and release of lysosomal enzymes. Loss of PIKfyve in platelets accelerates arterial thrombosis Platelets have long been known to contain primary lysosomes and release their lysosomal enzymes in response to stimuli [31] , [32] , but the physiologic role of platelet lysosome secretion has not been clearly delineated. Thus, we tested whether the lysosomal abnormalities observed in PIKfyve-null platelets correlated with any functional abnormalities. Washed platelets from control or PIKfyve fl/fl Pf4-cre mice formed aggregates to a similar degree in response to different agonists ( Supplementary Fig. 6e ), suggesting that activation of the dominant platelet integrin, αIIbβ3, is intact in the PIKfyve-null platelets. In addition, Akt phosphorylation was normally induced upon stimulation ( Fig. 5f ), suggesting that the intracellular signalling pathway in PIKfyve-null platelets is also preserved. To determine the effect of PIKfyve ablation in platelets during thrombosis in vivo , the carotid arteries of mice were analysed for occlusive thrombus formation in response to a chemical injury with ferric chloride. At 12–16 weeks of age, PIKfyve fl/fl Pf4-Cre mice formed occluding thrombi significantly faster than their control littermates (3.8±1.6 min versus 6.1±1.2 min, Fig. 5e ). Since PIKfyve-null platelets showed normal aggregation ex vivo , we speculated that the excessive secretion of the platelet lysosomal contents from PIKfyve-null platelets could contribute to endothelial damage and systemic inflammation leading to accelerated thrombus formation. Consistent with this possibility, plasma levels of vWF, a marker of endothelial damage and systemic inflammation [33] , were significantly elevated in the plasma of PIKfyve fl/fl Pf4-Cre mice when measured by immunoblotting ( Fig. 5g ) or enzyme-linked immunosorbent assay (ELISA; Fig. 5h ). Together, these results suggest that excessive lysosomal secretion from PIKfyve-null platelets is associated with endothelial damage and systemic inflammation, perhaps underlying excessive thrombosis in PIKfyve fl/fl Pf4-Cre mice. Impaired release of platelet lysosomes reverts the pathology If the pathological macrophage inflammatory response in PIKfyve fl/fl Pf4-Cre mice reflects the excessive stimulus-induced secretion of lysosomal enzymes, we hypothesized that attenuating the release of platelet lysosomes would comparably attenuate the inflammatory responses. To test this hypothesis, PIKfyve fl/fl Pf4-Cre mice were crossed with pallid mice, a model of Hermansky–Pudlak syndrome type 9 (ref. 34 ). Pallid mice lack an essential subunit of BLOC-1, a complex required for the biogenesis of lysosome-related organelles such as pigment cell melanosomes and platelet dense granules [35] , [36] . Importantly, stimulus-dependent secretion of lysosomal contents is impaired (but not ablated) in platelets from pallid mice [37] . In contrast to PIKfyve fl/fl Pf4-Cre mice that developed persistent dorsal alopecia and weight gain, PIKfyve fl/fl Pf4-Cre/pallid mice maintained hair growth until death and exhibited attenuated weight gain ( Fig. 6a,b ; note that because the pallid mutation also impairs melanosome biogenesis, pallid mice exhibit hypopigmented fur). As expected, platelet and plasma levels of β-hexosaminidase were lower in PIKfyve fl/fl Pf4-Cre/pallid mice than in PIKfyve fl/fl Pf4-Cre mice ( Fig. 6c,d ). Together, these data suggest that the release of platelet lysosomes contributes to the pathogenesis of multiorgan defects in PIKfyve fl/fl Pf4-Cre mice. 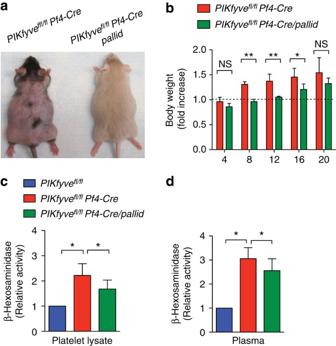Figure 6: Impaired secretion of platelet lysosomes attenuates the phenotypes ofPIKfyvefl/flPf4-Cremice. (a) General appearance ofPIKfyvefl/flPf4-Cremice andPIKfyvefl/flPf4-Cre/pallidmice on C57BL/6 background at 17 weeks of age. In the presence of thepallidmutation, the hair loss and weight gain are attenuated in thePIKfyvefl/flPf4-Cre/pallidmice. Note that thepallidmice have an underlying defect in melanosome biogenesis causing hypopigmented fur. (b) Body weight of thePIKfyvefl/flPf4-Cremice, and the sex-matched and age-matchedPIKfyvefl/flPf4-Cre/pallidmice. The average numbers of mice were five per time point and per group. The dashed line indicates the mean ratio of body weight of the control mice. (c,d) Analysis of β-hexosaminidase activity in the platelet lysate (c) and plasma (d) of thePIKfyvefl/flPf4-Cremice (n=3) and thePIKfyvefl/flPf4-Cre/pallid(n=3) mice. *P<0.05, **P<0.01. All error bars indicate mean±s.d. Student’st-test. Figure 6: Impaired secretion of platelet lysosomes attenuates the phenotypes of PIKfyve fl/fl Pf4-Cre mice. ( a ) General appearance of PIKfyve fl/fl Pf4-Cre mice and PIKfyve fl/fl Pf4-Cre/pallid mice on C57BL/6 background at 17 weeks of age. In the presence of the pallid mutation, the hair loss and weight gain are attenuated in the PIKfyve fl/fl Pf4-Cre/pallid mice. Note that the pallid mice have an underlying defect in melanosome biogenesis causing hypopigmented fur. ( b ) Body weight of the PIKfyve fl/fl Pf4-Cre mice, and the sex-matched and age-matched PIKfyve fl/fl Pf4-Cre/pallid mice. The average numbers of mice were five per time point and per group. The dashed line indicates the mean ratio of body weight of the control mice. ( c , d ) Analysis of β-hexosaminidase activity in the platelet lysate ( c ) and plasma ( d ) of the PIKfyve fl/fl Pf4-Cre mice ( n =3) and the PIKfyve fl/fl Pf4-Cre/pallid ( n =3) mice. * P <0.05, ** P <0.01. All error bars indicate mean±s.d. Student’s t -test. Full size image In this study, we show that PIKfyve kinase activity is critical in limiting the pathological inflammatory and thrombotic functions of platelet lysosomes. Our data indicate that PIKfyve kinase activity in platelets is essential for the normal maturation of cathepsin D and for the proper storage and release of lysosomal enzymes. Unexpectedly, dysregulated lysosomal homeostasis and enhanced lysosomal release from PIKfyve-null platelets drive an aberrant inflammatory response in macrophages. This leads to chronic inflammation and arterial thrombosis that affect the development, body mass, fertility and survival of mice. Our study shows that PIKfyve-null platelets excessively accumulate lysosomal components, which include lysosomal membrane proteins as well as lysosomal enzymes such as β-hexosaminidase and procathepsin D. Procathepsin D is targeted from the trans-Golgi network (TGN) to endosomes primarily via the mannose-6-phosphate receptor (M6PR) pathway and is further processed to active cathepsin D in acidic lysosomes [38] . The M6PR must then recycle to the TGN for another round of transport. The excessive accumulation and release of procathepsin D in PIKfyve-null platelets suggests that PIKfyve is critical for procathepsin D trafficking from the TGN to endosomes. This conclusion is consistent with a published study showing that PtdIns(3,5)P 2 deficiency leads to the defective retrograde trafficking of M6PR from endosomes to the TGN [39] , which would ultimately exhaust the M6PR from the TGN and result in default secretion of procathepsin D. Similarly, the fibroblasts of Vac14-null mice develop defective steady-state localization of M6PR, and they also accumulate the immature forms of cathepsin D [13] . Since PtdIns(3,5)P 2 is also required for acidification of the lysosome-like vacuole in yeast [9] and because the low pH in lysosomes is essential for the proteolytic maturation of procathepsin D [40] , an abnormal lysosomal pH could also contribute to the defective processing of procathepsin D in the PIKfyve-null platelets. In addition, wild-type platelets contain and secrete only minor amounts of procathepsin D whereas PIKfyve-null platelets excessively store and release procathepsin D. This suggests that PtdIns(3,5)P 2 deficiency might additionally feed back on lysosomal enzyme biosynthesis, perhaps by activating the CLEAR (coordinated lysosomal expression and regulation) gene network [41] , [42] . Interestingly, overexpression and secretion of procathepsin D have been found in several human cancers, including breast and lung carcinomas [43] . In these tumour cells, alterations of pathways that are M6PR dependent and independent have both been suggested [44] , [45] . In addition, excessive release of the lysosomal enzymes are also seen in the lysosomal storage disorders, Mucolipidosis II and Mucolipidosis III [46] . In these diseases, an inability to generate the M6P recognition signal on the lysosomal enzymes impairs their delivery from the TGN to the lysosome via the M6PR pathway resulting in the excessive release of lysosomal enzymes extracellularly [47] . Thus, the absence of PIKfyve in platelets results in a phenotype that is reminiscent of several human disorders with impaired trafficking from the TGN to the lysosome. Similar to PIKfyve deficiency, the deficiency of the inositol phosphatase and PIKfyve chaperone protein called Fig4 results in the reduced intracellular PtdIns(3,5)P 2 concentrations. Notably, Fig4-deficient mice develop enlarged endolysosomal vacuoles and excessive accumulation of lysosomal proteins, reminiscent of lysosomal storage diseases [48] . Likewise, mice lacking another PIKfyve-binding partner called Vac14 have decreased synthesis of PtdIns(3,5)P 2 and develop excessive vacuolation of late endosomal and lysosomal compartments [13] . Together with our findings, these studies further support that the depletion of PtdIns(3,5)P 2 by impairing any components of the PIKfyve complex could lead to the features that are reminiscent of those found in lysosomal storage disorders. It is notable that lysosomal storage diseases are frequently associated with inappropriate immune responses that result in chronic inflammation. For example, tissue infiltration of reactive macrophages can lead to visceral organomegaly in both Gaucher and Niemann-Pick diseases [49] , [50] . Likewise, microglial activation is frequently associated with the neuropathology in Mucopolysaccaridoses [51] . Similar to these findings, we unexpectedly observed that the ablation of PIKfyve in platelets causes inflammatory responses that are associated with robust macrophage defects, which lead to organomegaly in mice. Using several lines of evidence, we demonstrated that this macrophage phenotype is non-cell-autonomous, showing that PIKfyve-null platelets can induce aberrant responses in normal macrophages. Interestingly, this inflammatory response has not been described in mice lacking Fig4 or Vac14. This could be explained because these mice do not survive long enough to fully develop the robust tissue accumulation of macrophages seen in PIKfyve fl/fl Pf4-Cre mice. However, a similar non-cell-autonomous phenomenon has also been observed in Fig4-null mice, which have a neurodegenerative disorder [14] . The genetic restoration of Fig4 exclusively in the neuronal cells of Fig4-null mice not only reverts the dysfunctions of neuronal cells, but it also reverts the dysfunctions of the adjacent oligodendrocytes including hypomyelination and maturation defects [52] . Together with our findings, these studies indicate that the depletion of PtdIns(3,5)P 2 in a single cell type may have indirect implications in other cell types. Furthermore, they also show that our findings are consistent with the broad secondary defects shown in lysosomal storage disorders. Megakaryocytes and platelets have long been known to possess lysosomes that contain different hydrolases including proteases and glycosidases [31] , [53] . Upon platelet activation in vivo , platelets release not only alpha granules and dense granules, but they also release their lysosomal contents [54] . The physiopathological role of platelet lysosome secretion is not well understood. However, it has been speculated that the release of platelet lysosomal enzymes may be required for the remodelling of extracellular matrix during wound healing [55] . In addition, the pathological release of lysosomal enzymes may also cause the local injury of the vascular wall leading to atherosclerosis and the focal thickening of arteries [56] . Thus, proper regulation of the platelet lysosomal secretion would be essential to maintain a normal response to wound healing, and also to avoid the inflammatory and thrombotic defects that could result from the excessive platelet lysosomal secretion. Consistent with this concept, this study shows that the excessive storage and secretion of lysosomal enzymes from platelets lacking PIKfyve result in the accelerated arterial thrombosis and inflammation observed in PIKfyve fl/fl Pf4-Cre mice. Thus, our studies further support that the proper regulation of platelet lysosomal storage and secretion have a crucial role in limiting the proinflammatory and prothrombotic functions of platelets. Our study demonstrates the novel finding that PIKfyve kinase activity is a critical regulator of the lysosomal pathway in mouse platelets. This work also provides evidence that in addition to the effects mediated by the release of platelets alpha and dense granules, secretion of platelet lysosomes may be a previously unrecognized initiator of vascular damage and inflammatory responses. These findings could have important implications and applications in the diagnosis and in the design of novel targets for clinical disorders mediated by platelets. Animal models All animals were maintained on standard chow and tap water under specific pathogen-free conditions. All animal procedures were approved by the Institutional Animal Care and Use Committees at the University of Pennsylvania. Targeting of the PIKfyve gene was generated using C57BL6 mice (inGenious Targeting Laboratory). A bacterial artificial chromosome derived from C57BL/6 (RPCI23) genomic DNA was used to construct the targeting vector. The targeting vector was designed to excise exons 37 and 38 of the mouse PIKfyve gene that encodes the activation loop of the kinase domain. The 7.55-kb long homology arm extended 5′ to exon 37, and the 1.5-kb short homology arm extended 3′ to exon 38. A pGK-gb2 loxP/FRT neocassette was inserted on the 3′ side of exon 38, and the single loxP site was inserted at the 5′ side of exon 37. The resulting 10.6-kb fragment was subcloned into an ~2.4-kb backbone vector (pSP72, Promega) containing an ampicillin selection cassette to generate a final targeting construct of 14.8 kb. C57BL/6 embryonic stem cells (ES) were electroporated with targeting vectors. Clones resistant to the G418 antibiotic were selected and screened by Southern blot and PCR to identify recombinant ES clones. The selected clones were microinjected into C57BL/6 blastocysts. Resulting chimeras with black coat colour were mated with wild-type C57BL/6 mice to generate PIKfyve F1 heterozygous offspring. F1 heterozygous mice were crossed with a FLP transgenic mouse to excise the neomycin cassette that was flanked by FRT sites. The resulting F2 mosaic offspring were crossed with wild-type mice to generate F3 heterozygotes that were missing the neomycin cassette. F3 heterozygotes were crossed to generate mice carrying the PIKfyve -floxed allele ( PIKfyve fl ). PIKfyve fl/fl mice were crossed with transgenic mice expressing Cre recombinase under the control of the platelet factor 4 promoter (Pf4-Cre) to induce tissue-restricted Cre recombination in the megakaryocyte lineage. For some experiments, PIKfyve fl/fl mice were crossed with a B6;129S4- Gt(ROSA)26Sor tm1Sor /J ( Rosa26-LacZ ) reporter strain and then with a Pf4-Cre transgenic mouse. For other experiments, PIKfyve fl/fl mice were crossed with B6-Cg- Pldn pa /J ( pallid ) mice, and their offspring were paired with the Pf4-Cre transgenic mice to generate PIKfyve fl/fl Pf4-Cre/pallid mice. For all studies, both female and male mice were used. Sex-matched littermates were used as controls for all studies if not indicated otherwise. PCR genotyping Genomic DNA isolated from mouse tail biopsies was used to genotype mice by PCR. The recombinant ES cells were identified with 5′- CCAGAGGCCACTTGTGTAGC -3′ and A3: 5′- CAGCCAGTGCTCGCATACAAAGG -3′ primers. The insertion of neomycin cassette in F1 mice was identified with 5′- CCAGAGGCCACTTGTGTAGC -3′ and 5′- GGATGAAGTGCCTTGTTATCTGCAG -3′ primers. The 3rd LoxP integration was identified with 5′- CCATTGCCTGGCTTAGAACAGAG -3′ and 5′- GAACTCTCCCGCGTAGTACAGC -3′ primers. PCR-generated products were either 310 bp corresponding to the wild-type alleles or 370 bp corresponding to the targeted allele (LoxP integrated). Pf4-Cre transgene was identified with 5′- CCCATACAGCACACCTTTTG -3′ and 5′- TGCACAGTCAGCAGGTT -3′ primers. Rosa26/LacZ transgene was identified with 5′- AAAGTCGCTCTGAGTTGTTAT -3′, 5′- GCGAAGAGTTTGTCCTCAACC -3′ and 5′- GGAGCGGGAGAAATGGATATG -3′. Body composition analysis Mice were anaesthesized with sodium pentobarbital (90 mg kg −1 ) and scanned by dual-energy X-ray absorptiometry at the Mouse Metabolism Core at the University of Pennsylvania. Histochemistry and immunohistochemistry Necropsies were performed on female and male control and PIKfyve fl/fl Pf4-Cre mice between 3 weeks and 28 weeks of age. They included macroscopic observations, body and organ weight measurements, complete blood counts, serum chemistry analysis and microscopic examination of the brain, thymus, lymph nodes, heart, lung, small intestine, large intestine, liver, spleen, pancreas, kidney, ovaries, testis, skin, muscle, fat and bone marrow. Fresh postmortem tissues were fixed overnight in 10% formalin, paraffin-embedded and sectioned. Paraffin sections were deparaffinized with xylene and ethanol, and stained with haematoxylin/eosin, periodic acid Schiff and Alcian blue. For immunohistochemistry, paraffin sections were deparaffinized with xylene and ethanol, and antigen retrieved in 0.01 M citrate buffer by microwaving for 30 min. They were stained with the following primary antibodies: F4/80 (Serotec; 1:100), CD41 (BD Pharmingen; MWReg30; 1:50) and CD45R/B220 (BD Pharmingen; RA3-6B2; 1:500). Sections were counterstained with haematoxylin. For X-gal staining, frozen tissue sections were fixed with 0.5% glutaraldehyde for 10 min, and stained overnight with the chromogenic substrate for β-galactosidase, X-gal (Cell Center, University of Pennsylvania). Sections were then counterstained with haematoxylin or haematoxylin/eosin as indicated. Immunoblotting Tissues were harvested and homogenized in RIPA buffer with a protease inhibitor cocktail (Roche). The protein concentrations were determined using the BCA Protein Assay (Pierce). Proteins were separated on SDS–PAGE gradient gels (Invitrogen) and then transferred onto the polyvinylidene difluoride membrane (Invitrogen). The membrane was blotted with the indicated primary antibodies against: PIKfyve-N-terminal (Sigma-Aldrich; P0054; 1:400), LAMP-1 (Developmental Studies Hybridoma Bank; 1:1,000), EEA-1 (Santa Cruz; 1:1,000), Cathepsin D (Calbiochem; 1:1,000), vWF (DAKO; 1:1,000), PF4 (Bethyl; 1:1,000), Akt (Cell Signaling Technology; 1:1,000), pAkt (Cell Signaling Technology; 1:1,000) and β-actin (Cell Signaling Technology; 1:1,000). This was followed by blotting with horseradish peroxidase-conjugated secondary antibodies and developing with enhanced chemiluminescence substrate (GE Healthcare). Full blots are shown in the Supplementary Figs 8 and 9 . Megakaryocyte and platelet preparation Megakaryocytes were derived from the bone marrow by flushing mouse femurs and cultured in the presence of 1% thrombopoietin (TPO, R&D Systems) in IDMD supplemented with 10% FBS [26] . After 4 days, cultured megakaryocytes were isolated by sedimentation through a 1.5%/3% BSA step gradient. To prepare washed platelets, blood was collected from the inferior vena cava of mice into 0.1 volume of acid citrate dextrose buffer. Platelet-rich plasma was separated by centrifugation at 200 g for 10 min and incubated with 1 μM prostaglandin E1 for 10 min at room temperature. Platelets were then isolated by centrifugation at 800 g for 10 min and resuspended in HEPES-Tyrode buffer pH 7.4. Megakaryocyte number and ploidy analysis To measure the number of megakaryocytes in the bone marrow, isolated megakaryocytes from the bone marrow were stained with CD41 antibody conjugated with Alexa 488 (BD Biosciences), and cells were counted on the FACS Calibur flow cytometer (BD Biosciences) discriminating size to subtract out platelets. To determine the megakaryocyte ploidy, cells were stained with propidium iodide (Sigma) and the relative DNA content was measured. FlowJo software was used to analyse all flow cytometry data. P-selectin expression analysis Platelets were diluted to a density of 5 × 10 6 cells ml −1 , stimulated with thrombin at indicated concentrations and then incubated with a phycoerythrin-conjugated P-selectin antibody (BD Pharmingen). Fluorescence values were analysed on a FACS Calibur flow cytometer (BD Biosciences). Platelet aggregation and ATP secretion Platelets were diluted to a density of 2.5 × 10 6 cells ml −1 in HEPES-Tyrode buffer pH 7.4. Platelet aggregation in response to agonist stimulation was assessed by changes in light transmission detected by a dual-channel lumi-aggregometer (Chrono-Log) with stirring at 37 °C. Platelet secretion of ATP was assessed concurrently by the luciferin/luciferase reaction after adding chrono-lume no. 395 (Chrono-Log) to the aggregometer cuvette. Transmission electron microscopy Megakaryocytes grown in culture were harvested on day 6 and fixed in glutaraldehyde. Ultrathin sections were obtained and collected on hexagonal copper grids. Sections were stained with Reynold’s lead citrate and examined using transmission electron microscopy at the Electron Microscopy Core Facility at the University of Pennsylvania. Platelet depletion in vivo To study the effects of platelet depletion in the control mice and the PIKfyve fl/fl Pf4-Cre mice, female and male mice at 8–10 weeks of age were administered with GPIbα antibody (Emfret) at 2 μgg −1 twice weekly by intraperitoneal injections for a total of 6 weeks. Blood counts were monitored weekly by collecting blood from the retro-orbital sinus. Body weight was monitored twice weekly. Necropsies were performed at the completion of 6 weeks of antibody treatment. Radiation bone marrow chimeras Bone marrow cells were isolated from wild-type mice expressing either CD45.1 or CD45.2 congenic markers or from PIKfyve fl/fl Pf4-Cre mice expressing CD45.2 congenic markers. Bone marrow cells were depleted of T cells and red blood cells by using magnetic beads bound to antibodies against Ter119, CD3, CD4 and CD8. To study the phenotype rescue effect, PIKfyve fl/fl Pf4-Cre recipient mice expressing CD45.2 congenic markers were irradiated with 900 rads and administered by retro-orbital injection with 2 × 10 6 bone marrow cells from wild-type mice expressing CD45.1 markers. To study the phenotype transfer effect, wild-type recipient mice expressing CD45.1 markers were irradiated with 900 rads, and administered by retro-orbital injection with 1 × 10 6 bone marrow cells from wild-type mice expressing thy 1.1 marker and 1 × 10 6 bone marrow cells from PIKfyve fl/fl Pf4-Cre mice expressing CD45.2 markers. Transplanted mice were maintained in sterile water with sulfamethoxazole/trimethoprim for 3 weeks. Mice were killed and analysed for engraftment and histology analyses at about 33–35 weeks after transplantation. β-Hexosaminidase and cathepsin D activity assays The β-hexosaminidase activity,was determined using a chromogenic substrate [57] . Mouse platelets or plasma were mixed with 10 mM substrate p -nitrophenyl- N -acetyl-β- D -glucosaminide (Sigma) in citrate-phosphate buffer pH 4.5. Platelet extracts were incubated for 16 h at 37 °C and plasma was incubated for 1 h at 37 °C. The enzymatic reaction was stopped by the addition of 0.5 M NaOH. The absorbance of released p-nitrophenolate was read at 405 nm in an ELISA plate reader. Cathepsin D activity was determined using a fluorogenic substrate [58] . The reaction mixture contained 10 μl of platelet lysate solution, 10 μl of 200 μM of substrate Bz-Arg-Gly-Phe-Phe-Pro-4MeOβNA (Calbiochem) and 80 μl of 50 mM sodium acetate buffer pH 4.0. Reaction mixtures were incubated for 30 min at 37 °C. The enzymatic reaction was stopped by adding 5% trichloroacetic acid. The release of 2-naphthylamine was measured in a spectrofluorometer at emission wavelength of 410 nm and excitation wavelength of 335 nm. FeCl 3 -induced carotid artery thrombosis assay Mice were anaesthetized using sodium pentobarbital (90 mg kg −1 ). A midline incision was made in the neck, and the carotid artery was exposed and dissected away from surrounding tissue. The artery was placed on a Doppler flow probe (Transonic Systems, Ithaca, NY) to monitor blood flow through the vessel. After a baseline flow measurement was recorded, vascular injury was initiated by placing a 1 mm 2 piece of filter paper saturated with 7.5% FeCl 3 (Sigma) on the surface of the artery for 2 min. The filter paper was then removed and the artery rinsed with saline, followed by the continuous recording of blood flow in the vessel for 20 min post injury. The time to vessel occlusion was recorded. Plasma vWF analysis For analysis of plasma vWF multimer distribution, mouse plasma (10 μl) was denatured at 60 °C for 20 min with 10 μl of sample buffer (70 mM Tris, pH 6.8, 2.4% SDS, 0.67 M urea, 4 mM EDTA, 10% glycerol, 0.01% bromophenol blue). Proteins were fractionated on 1% agarose gel on ice and transferred to a nitrocellulose membrane. The membrane was blotted with vWF IgG antibody (Dako; 1:5,000) to detect the vWF multimers. For quantification analysis of plasma vWF antigen, we performed ELISA. A microtitre plate coated with rabbit anti-vWF IgG (Dako; 1:2,000) was incubated with diluted mouse plasma for 1 h at room temperature. After washing with phosphate-buffered saline, bound vWF was determined by peroxidase-conjugated rabbit anti-vWF IgG (Dako; 1:2,000). A pre-mixed TMB (3,3′,5,5′-tetramethylbenzidine) solution was used for colour development. The absorbance at 450 nm was determined by an ELISA plate reader. Mass spectrometry analysis To prepare platelet releasates for proteomics analysis, washed platelets (5 × 10 8 cells ml −1 ) were stimulated with 1 U ml −1 thrombin for 10 min at 37 °C. Activated platelets were centrifuged at 13,000 g for 10 min at 4 °C and the supernates were isolated from the pellets. The concentrations of proteins from the platelet supernates were measured using the BCA protein assay (Pierce). Proteins (40 μg) were digested with trypsin in solution. Tryptic digests were analysed by LC-MS/MS on a hybrid LTQ-Orbitrap Elite mass spectrometer (Thermofisher Scientific, San Jose, CA) coupled with a nano LC Ultra (Eksigent). Peptides were separated by reverse phase (RP)-HPLC on a nanocapillary column, 75 μm id × 15 cm Reprosil-pur 3 μM (Dr Maisch, Germany) in a Nanoflex chip system (Eksigent). Mobile phase A consisted of 1% methanol (Fisher)/0.1% formic acid (Thermo) and mobile phase B of 1% methanol/0.1% formic acid/80% acetonitrile. Peptides were eluted into the mass spectrometer at 300 nl min −1 with each RP-LC run comprising a 90 min gradient from 10 to 25% B in 65 min, 25–40% B in 25 min. The mass spectrometer was set to repetitively scan m / z from 300 to 1,800 ( R =240,000 for LTQ-Orbitrap Elite) followed by data-dependent MS/MS scans on the twenty most abundant ions, with a minimum signal of 5,000, dynamic exclusion with a repeat count of 1, repeat duration of 30 s, exclusion size of 500 and duration of 60 s, isolation width of 2.0, normalized collision energy of 33 and waveform injection and dynamic exclusion enabled. FTMS full scan AGC target value was 1e6, while MSn AGC was 1e4, respectively. FTMS full scan maximum fill time was 500 ms, while ion trap MSn fill time was 50 ms; microscans were set at 1. FT preview mode; charge state screening and monoisotopic precursor selection were all enabled with rejection of unassigned and 1+ charge states. For database search, MS/MS raw files were searched against a mouse protein sequence database including isoforms from the Uniprot Knowledgebase (taxonomy:10090 AND keyword: ‘Complete proteome [KW-0181]’) using MaxQuant version 1.4.1.2 with the following set parameters: fixed modifications, Carbamidomethyl (C); decoy mode, revert; MS/MS tolerance ITMS, 0.5 Da; false discovery rate for both peptides and proteins, 0.01; minimum peptide length, 6; modifications included in protein quantification, acetyl (protein N-term), oxidation (M); peptides used for protein quantification, razor and unique. The numbers of peptide spectral matches to each protein were used for quantitative comparison between samples as described below. For statistical analysis of mass spectrometry data, we adapted a method proposed by Choi [59] to use the number of peptide spectral matches (PSMs) in each protein to determine the likelihood that the protein was differentially regulated across the control mice and the knockout mice. The idea is to develop a control model and a knockout model, and, for each protein, to test whether the knockout model describes its expression data significantly better than the control model. To do so, we estimate a Bayes Factor for each protein. We assume that the number of PSMs for protein p in sample i can be modelled as a Poisson distribution with mean λ pi , since each element x pi in the data matrix X is count data. To combat the limited number of biological replicates in each treatment group, we pooled information across replicates and estimate each λ pi using a control and knockout hierarchical log-linear model, denoted by: where L p is the length of protein p , N i is the mean number of spectral counts in sample i , a 0 is a model constant, c p is a protein’s native expression term and k p is a protein’s knockout expression term. We give the model a well-defined structure by putting priors on a 0 ~ N (0, δ a 2 ), c p ~ N (0, δ c 2 ), and k p ~ N (0, δ k 2 ). To make data-driven estimates of δ c 2 and δ k 2 , we place hyper priors on these two parameters, given by δ c 2 , δ k 2 ~InvGamma(0.1, 0.1). We let a 0 ‘float’, and thus set δ a 2 =10 2 . We use these parameters (denoted as a vector by θ ) to estimate a protein’s Bayes Factor: where the transition states are determined using Metropolis Hastings and Gibbs Sampling Markov Chain Monte Carlo techniques. Specifically, at iteration n with parameter vector θ K (we explain using the knockout model, since M C ⊂ M K ), where G is the number of proteins. To determine the set of proteins that significantly changed in the knockout set with respect to the control set, we imposed a strict cutoff and the requirement that each protein have a Bayes Factor of at least 8 and a fold change of at least 2.0. Statistical analysis GraphPad Prism 5 was used to analyse data. All data are presented as mean±s.d. Two-tailed Student’s t -tests were used for the comparison of two groups. A log-rank test was performed for Kaplan–Meier survival analysis. P -values of <0.05 (*), <0.01 (**) and <0.001 (***) were used to ascertain statistical significance. How to cite this article: Min, S. H. et al . Loss of PIKfyve in platelets causes a lysosomal disease leading to inflammation and thrombosis in mice. Nat. Commun. 5:4691 doi: 10.1038/ncomms5691 (2014).